Insights into the role of DNA methylation in diatoms by genome-wide profiling inPhaeodactylum tricornutum DNA cytosine methylation is a widely conserved epigenetic mark in eukaryotes that appears to have critical roles in the regulation of genome structure and transcription. Genome-wide methylation maps have so far only been established from the supergroups Archaeplastida and Unikont. Here we report the first whole-genome methylome from a stramenopile, the marine model diatom Phaeodactylum tricornutum . Around 6% of the genome is intermittently methylated in a mosaic pattern. We find extensive methylation in transposable elements. We also detect methylation in over 320 genes. Extensive gene methylation correlates strongly with transcriptional silencing and differential expression under specific conditions. By contrast, we find that genes with partial methylation tend to be constitutively expressed. These patterns contrast with those found previously in other eukaryotes. By going beyond plants, animals and fungi, this stramenopile methylome adds significantly to our understanding of the evolution of DNA methylation in eukaryotes. DNA cytosine methylation (m5C) is a conserved epigenetic modification in eukaryotes, involved in several important biological processes such as silencing of transposable elements (TEs) and other repeat loci [1] , X chromosome inactivation in female mammals [2] , parent-of-origin genomic imprinting [3] and the regulation of gene expression [4] . Recently, whole-genome methylomes have been reported from a range of plants, fungi and animals. These have shown that in addition to the methylation found in TEs and other repeat sequences, the presence of m5C in the bodies of genes also appears to be common in many eukaryotic genomes [5] , [6] , [7] , [8] , [9] , [10] . In most organisms, the presence of m5C in repeat loci represents the primary mechanism of TE suppression, whereas there is no known specific function of intragenic methylation. In addition to revealing common aspects of eukaryotic methylation systems, these previous studies have also shed light on the highly variable evolution of m5C functions, patterns and landscapes across eukaryotic groups and lineages. For example, transcriptionally silent repeat loci have been observed to be hypomethylated in invertebrates [9] , [10] , [11] , suggesting that m5C may not be involved in TE suppression in these organisms. Conversely, genes from the early-diverging vascular plant Selaginella moellendorffii and the moss Physcomitrella patens contain only trace levels of m5C compared with those found in angiosperms [10] , underlying the variability of DNA methylation among living organisms. In fungi, m5C is concentrated in repeat loci whereas active genes are not methylated [6] , [9] . Furthermore, several model eukaryotes are devoid of DNA methylation altogether, including the yeast Saccharomyces cerevisiae [12] , the nematode Caenorhabditis elegans [13] , the fruit fly Drosophila melanogaster [14] (except in the early stages of embryogenesis [15] ) and the brown alga Ectocarpus siliculosus [16] . From the methylomes examined thus far, it is therefore unclear which are the ancestral underlying mechanisms at work and those that have been co-opted to distinct biological roles in different eukaryotic groups. To address such evolutionary issues, a more thorough exploration of the distribution of cytosine methylation throughout the genomes of a wider range of eukaryotes is required. To date, all the whole-genome methylomes that have been reported are from two major eukaryotic groups: Unikont and Archaeplastida [17] ( Supplementary Fig. S1 ). Stramenopiles, on the other hand, represent a major lineage of eukaryotes that appeared following a secondary endosymbiosis event involving a heterotrophic exosymbiont host and algal endosymbionts [18] , [19] . Among these, diatoms constitute a highly successful and diversified group, with possibly over 10,000 extant species. The contribution of diatoms to marine primary productivity has been estimated to be around 40% and they have a key role in the biological carbon pump as well as a major resource at the base of the food chain [18] . P. tricornutum has become an attractive model diatom because of the availability of genetic tools and a fully sequenced genome [20] , [21] . It contains a range of genes with characterized evolutionary histories [19] , [20] , and in addition to genes of exosymbiont and algal endosymbiont origins, comparative analyses suggest that a significant number of genes (>500) are most closely related to genes of bacterial origin [20] . The genome also contains a diverse set of DNA methyltransferases (DNMTs) [22] . P. tricornutum can therefore be used to probe the evolutionary history of DNA methylation, and to ask whether genes of different origins have maintained distinctive epigenetic marks. In this report, we combine McrBC digestion with whole-genome tiling array hybridization, DNA bisulphite sequencing and RNA sequencing to address the genome-wide distribution of methylation and its potential role in genome regulation and control of transcription in P. tricornutum . Whole-genome methylation landscape Methylated and unmethylated DNA from P. tricornutum were fractionated following a protocol based on the exclusion of methylated DNA by digestion with the methyl-sensitive endonuclease McrBC [23] . After whole-genome amplification, the samples were hybridized to a high-definition tiling array of the P. tricornutum genome (McrBc-chip; see Methods ). We found a total of 98,080 probes out of ~2.2 million on the array with significant enrichment probability, which we further clustered into ‘highly methylated regions’ (HMRs) that we arbitrarily defined as loci with at least three overlapping enriched probes. We purposely chose this conservative cutoff in order to reduce falsely identified regions and to focus on the most significant signals in our analysis. Only these HMRs were used for further analysis. Genomic features were then considered methylated if they overlapped with an HMR. We validated our methylation mapping approach by bisulphite sequencing of 76 randomly chosen loci including genes and TEs that are distributed at different locations in the genome ( Supplementary Tables S1, S2 and S3 , Supplementary Fig. S2 ). These analyses revealed highly similar methylation patterns compared with the array analysis, validating further the cutoff chosen for defining HMRs. From these analyses, 5mC was found in the sequence context of CG, CHG and CHH (where H can be any nucleotide other than G). However, most of the methylation is found in a CG context ( Supplementary Fig. S3a ). We detected 3,887 HMRs that together cover 1,412,473 base pair (bp) (~5.16%) of the 27.4-Mb P. tricornutum nuclear genome ( Supplementary Table S4 ). The length of HMRs ranged from 60–5,700 nucleotides, the majority being shorter than 500 bp ( Supplementary Fig. S3b ). We used HMRs to construct a methylation map for each P. tricornutum genomic scaffold ( Supplementary Fig. S4 ). As expected, we observed extensive DNA methylation in repeat-rich regions (39% of such sequences), including in subtelomeric regions, although no obvious centromeric regions could be detected, neither at DNA sequence level nor in terms of DNA methylation enrichment ( Supplementary Fig. S4 ). We also found a significant number of HMRs in repeat-free regions. A total of 587 HMRs mapped to intergenic regions, whereas 505 HMRs mapped within predicted genes (including 500 bp upstream and downstream of predicted gene bodies). In addition, 604 HMRs mapped to predicted genes that overlap with TE annotations. For further analysis, such genes ( n =766) were omitted from the regular gene set and considered as a distinct annotation class in order to circumvent a bias due to erroneous gene predictions at TE loci and to focus on the most reliable gene predictions. HMRs in TEs and other repeat loci We first characterized HMRs mapping within known autonomous TEs. The P. tricornutum TE complement consists principally of LTR retrotransposons (CoDis) and a few copies of DNA transposons, including PiggyBac and Mutator-like elements [24] . We observed heterogeneous distribution of DNA methylation across the different groups of TEs ( Fig. 1 ). For example, while most LTR-RT annotations contain HMRs, a significant fraction of Mutator-like annotations do not ( Fig. 1a ). Furthermore, we observed that TE annotations corresponding to LTR-RT elements are extensively methylated, while those corresponding to DNA transposons are methylated to a lesser extent ( Fig. 1a ). In parallel, we noticed that the coverage and presence of HMRs increase linearly with the length of TE annotations ( Fig. 1b ). These observations might be due to a tighter control of potentially active TE copies, especially against CoDis, which were recently amplified in this genome [24] ( Fig. 1b ). 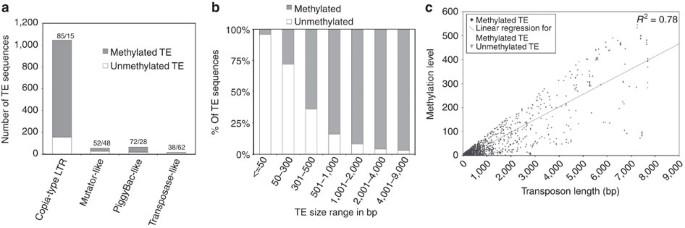Figure 1: DNA methylation in TEs. (a) Number of methylated sequences and methylation coverage for different types of TEs (only for TE annotations above 300 bp). Percentage of methylated TEs in each class is shown for each of the four classes. (b) Proportion of methylated sequences across size ranges of TEs and other repeats. (c) Plot of the methylation level versus TE length. Methylation level is the sum of enriched probes in the annotation. A total of 1,368 TEs and repeat sequences were found to be methylated (39%). Figure 1: DNA methylation in TEs. ( a ) Number of methylated sequences and methylation coverage for different types of TEs (only for TE annotations above 300 bp). Percentage of methylated TEs in each class is shown for each of the four classes. ( b ) Proportion of methylated sequences across size ranges of TEs and other repeats. ( c ) Plot of the methylation level versus TE length. Methylation level is the sum of enriched probes in the annotation. A total of 1,368 TEs and repeat sequences were found to be methylated (39%). Full size image We next addressed the distribution of HMRs in the 766 predicted genes that overlap with TE annotations. We sorted these into two categories: genes with partial TE coverage that may correspond to genes with TE insertions, and genes with complete TE coverage that may correspond to TE loci misannotated as genes. As for TEs, we observed that most ‘genes’ with complete TE coverage contain HMRs ( Supplementary Fig. S5 ) and manual examination confirmed that they indeed represent bona fide TEs. By contrast, most of the genes with internal TE insertions do not contain HMRs localized to the TE homologous region, suggesting that they may correspond to old insertions or that TE methylation may be suppressed in the case of intragenic insertions (especially within introns; see below). Gene methylation profiles The 505 HMRs mapping within genes were distributed in the bodies and flanking 500 bp sequences of 326 genes, among which 298 were confirmed to be methylated by bisulphite sequencing. A positive correlation between the output of the two methods is shown in Supplementary Fig. S6 . As found in most eukaryotes examined to date, methylation in the body of P. tricornutum genes occurs almost exclusively in exons ( Supplementary Fig. S7 ). Interestingly, we found that although most P. tricornutum genes contain 1–2 exons, methylated genes tend to contain more exons than unmethylated genes ( Supplementary Fig. S8 ). In addition, although highly methylated genes are typically single exon genes, the few P. tricornutum genes with five or more exons show higher methylation levels than those with 3–4 exons ( Supplementary Fig. S8b ). Furthermore, the size distribution of methylated genes is skewed towards longer genes as compared with unmethylated genes, that is, the frequency of methylated genes longer than 2 kb is higher than that of unmethylated genes (Welch two sample t -test P -value=3.612e−06) ( Supplementary Fig. S8c ). Overall then, methylated genes in P. tricornutum tend to be longer and to contain more exons than unmethylated genes. Analysis of genic regions shows that, on average, methylation levels increase from 5′ to 3′ within the gene body (defined as everything that is between the ATG and the stop codon) with sharp reductions at the ends ( Fig. 2 ). Such a pattern is most similar to that observed in the bodies of Arabidopsis, mammalian and fish genes, and is in contrast to what has been described in the genomes of most invertebrates where methylation is found predominantly within the first half of the coding sequence [5] , [6] , [10] . 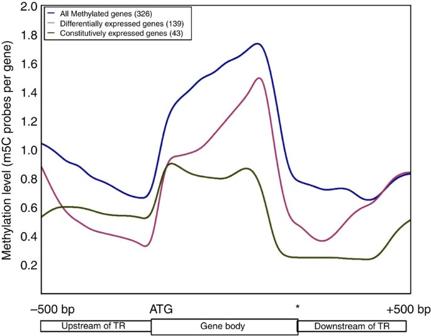Figure 2: Methylation profiles of genes. DNA methylation pattern is shown along gene bodies and 500 bp gene-flanking regions. A moving window of 50 bp along the sequence was used to calculate the average number of m5C probes (yaxis). Gene methylation profiles with respect to their expression is also shown. Constitutively expressed genes display low methylation levels along their transcribed sequence, whereas differentially expressed genes have an overall higher and increasing methylation level from 5′- to 3′-end of genes. * indicates the stop codon and TR the transcribed region. Figure 2: Methylation profiles of genes. DNA methylation pattern is shown along gene bodies and 500 bp gene-flanking regions. A moving window of 50 bp along the sequence was used to calculate the average number of m5C probes ( y axis). Gene methylation profiles with respect to their expression is also shown. Constitutively expressed genes display low methylation levels along their transcribed sequence, whereas differentially expressed genes have an overall higher and increasing methylation level from 5′- to 3′-end of genes. * indicates the stop codon and TR the transcribed region. Full size image We further distinguished several patterns of DNA methylation in genes: extensive methylation from upstream to downstream, as well as partial methylation, which we subdivided into categories following the position of the methylation peak: upstream 500 bp, 5′-end of gene body (relative first 20% of gene body), middle of gene body, 3′-end of the gene body (relative last 20% of gene body) and downstream 500 bp. The 500 bp region upstream of the start codon was defined as putative promoter region, as the intergenic length in P . tricornutum varies between 1,000 and 1,500 bp. We found that intragenic methylation occurs for 173 genes in the mid-gene body region while relatively few methylation profiles peak in the 5′- or 3′-ends ( Supplementary Table S5 , Fig. 2 ). We also noticed a substantial number of genes with the highest levels of methylation in their promoters. Besides these, we detected 25 genes with extensive methylation throughout. Methylation appears to be distributed evenly among genes belonging to different orthology groups, previously defined by Bowler et al . [20] and Maheswari et al . [25] as being present either in all eukaryotes, as being P. tricornutum -specific or diatom-specific, or predicted to have been acquired from bacteria by horizontal gene transfer ( Supplementary Fig. S9 ). Notwithstanding, bacterial genes are less likely to be methylated ( P -value=0.0001, Student t -test). However, the most strongly methylated genes appear to be depleted in P. tricornutum -specific genes and eukaryotic core genes, and rather to be enriched in other genes with unclear phylogenetic affiliations ( P -value=0.0001, Student t -test, Supplementary Fig. S9 ). Genomic distribution of methylated genes In order to analyse the chromosomal distribution of body-methylated genes, they were mapped onto the P. tricornutum scaffolds and their positions were compared with TE annotations. We observed that body-methylated genes are found in different genomic contexts. First, we found that 149 methylated genes are located in the vicinity of TEs (for example, Fig. 3a ). A more detailed analysis indeed revealed that methylated genes are often located close to TEs ( Fig. 4 ). Considering that TEs are in most cases extensively methylated in the genome, we postulate that DNA methylation in such genes may result by spreading from TEs, as reported in Arabidopsis thaliana [26] . This suggests that TE insertion followed by DNA methylation may impact the epigenetic status and expression levels of flanking genes (see below). However, not all TE-flanking genes are methylated ( Fig. 3b ), suggesting that spreading, or its avoidance, is a selective process. In repeat-free regions, we found that methylated genes are isolated ( Fig. 3d ) or juxtaposed to one another in clusters comprising 2–3 genes (for example, Fig. 3e ). 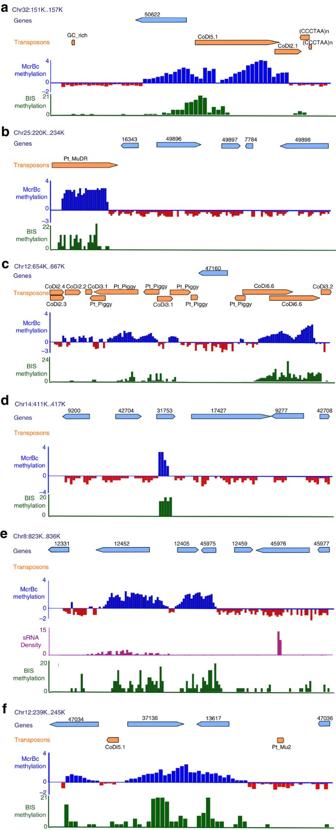Figure 3: Methylation patterns of selected genes. Four tracks (genes, transposons, McrBc and bisulphite methylation) along with chromosome position are shown for each example. (a) Region on chromosome 32 containing a methylated gene bordering a cluster of methylated TEs. (b) Region on chromosome 25 containing methylated TEs with a cluster of nonmethylated genes. (c) Region on chromosome 12 containing a nonmethylated bacterial gene (ID 47160) surrounded by methylated TEs. (d) Example of highly methylated gene. (e) Example of highly methylated gene cluster. Region on chromosome 8, isolated from methylated TEs, containing a cluster of methylated genes. Note that gene 12452, encoding a P-type ATPase, is also targeted by small RNAs (data from Huanget al.42). (f) Example of highly methylated gene displaying strong differential expression. Under normal conditions, gene 13617 (encoding a serine/threonine protein kinase) is methylated with no expression but expressed specifically under silicate-deplete conditions25. Heights of the peak represent the normalized log ratio (score) of the m5C probes. Genes and TE annotations are indicated. Figure 3: Methylation patterns of selected genes. Four tracks (genes, transposons, McrBc and bisulphite methylation) along with chromosome position are shown for each example. ( a ) Region on chromosome 32 containing a methylated gene bordering a cluster of methylated TEs. ( b ) Region on chromosome 25 containing methylated TEs with a cluster of nonmethylated genes. ( c ) Region on chromosome 12 containing a nonmethylated bacterial gene (ID 47160) surrounded by methylated TEs. ( d ) Example of highly methylated gene. ( e ) Example of highly methylated gene cluster. Region on chromosome 8, isolated from methylated TEs, containing a cluster of methylated genes. Note that gene 12452, encoding a P-type ATPase, is also targeted by small RNAs (data from Huang et al . [42] ). ( f ) Example of highly methylated gene displaying strong differential expression. Under normal conditions, gene 13617 (encoding a serine/threonine protein kinase) is methylated with no expression but expressed specifically under silicate-deplete conditions [25] . Heights of the peak represent the normalized log ratio (score) of the m5C probes. Genes and TE annotations are indicated. 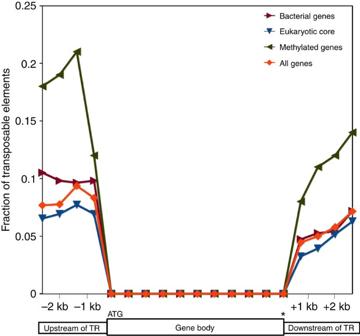Figure 4: Distribution of TEs around genes. The plot shows TE distribution within 2 kb upstream and downstream of all genes (n=10,408), bacterial genes (n=571), methylated genes (n=326) and eukaryotic genes (n=2,775). Clusters of TEs within the 2 kb region upstream of bacterial genes were more common than the other classes. * indicates the stop codon and TR the transcribed region. Full size image Figure 4: Distribution of TEs around genes. The plot shows TE distribution within 2 kb upstream and downstream of all genes ( n =10,408), bacterial genes ( n =571), methylated genes ( n =326) and eukaryotic genes ( n =2,775). Clusters of TEs within the 2 kb region upstream of bacterial genes were more common than the other classes. * indicates the stop codon and TR the transcribed region. Full size image We next analysed the distribution of TEs and repeat sequences in the vicinity of genes previously defined as being present in all eukaryotes, or predicted to have been acquired from bacteria by horizontal gene transfer [20] , [25] . Interestingly, we noticed an increased presence of TEs around putative bacterial genes ( Fig. 4 ), represented by gene IDs 16343 and 47160 in Fig. 3b , respectively. In spite of this, the proportion of methylated bacterial genes in the genome was less than in other gene categories ( Supplementary Fig. S9 ) suggesting that TEs do not necessarily induce bacterial gene methylation by spreading or making the genomic region where they are inserted prone to methylation. DNA methylation and gene expression To assess whether gene (includes gene body plus upstream and downstream 500 bp) methylation impacts transcriptional regulation in P. tricornutum , we compared the expression levels of methylated versus unmethylated genes. Expression levels were quantified using RNA-seq data obtained from P. tricornutum cells grown under normal conditions, and normalized to coding sequence length and library size (fragments per kilobase of exon per million fragments mapped, FPKM). We analysed separately the genes with different HMR peak locations and genes with extensive HMR coverage. Interestingly, while genes with partial intragenic methylation displayed expression levels similar to unmethylated genes, those with extensive HMR coverage show on average a markedly lower FPKM ( Fig. 5a ). In analogy with Ascobulus immersus [27] , such a negative correlation between the extent of methylation and gene expression levels suggests a suppressive role for extensive gene methylation. We also observed that methylation in the promoter (upstream 500 bp) of genes does not appear to impact transcription levels. 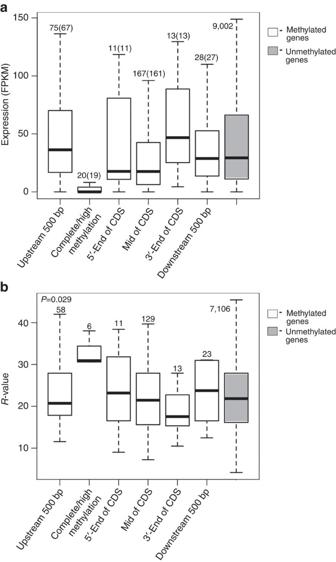Figure 5: Expression profiles of methylated genes. (a) Expression levels of methylated genes. Gene expression was quantified in standard growth conditions using RNA-seq data. About 85% of genes are expressed and quantified as fragments per kilobase of exons per million reads mapped (FPKM). Highly methylated genes have the lowest expression level compared with the other categories. Unmethylated genes have similar expression pattern than the genes falling into the upstream and downstream 500 bp categories. The number of genes confirmed as being methylated by bisulphite sequencing (seeMethods) is also indicated between parentheses. Extensively methylated genes are the ones that have HMR from 500 bp upstream of 5′-end to 500 bp downstream of 3′-end. (b) Differential expression profiles of methylated genes. Boxplots show the ranges ofR-values for each category of methylated genes. Genes withR-values below 12 are considered to be constitutively expressed25. Of the 20 densely methylated genes, a total of six were defined as being differentially expressed (P-value of 0.029, Studentt-test). Another seven genes were expressed in normal growth conditions (shown by RNA-seq data) whereas the remaining sevenbona fidegenes were not expressed in any of the tested conditions. Medians of the data are shown as black horizontal line in the box. Outliers are shown as whiskers. Numbers above each column show the number of genes in each category. Figure 5: Expression profiles of methylated genes. ( a ) Expression levels of methylated genes. Gene expression was quantified in standard growth conditions using RNA-seq data. About 85% of genes are expressed and quantified as fragments per kilobase of exons per million reads mapped (FPKM). Highly methylated genes have the lowest expression level compared with the other categories. Unmethylated genes have similar expression pattern than the genes falling into the upstream and downstream 500 bp categories. The number of genes confirmed as being methylated by bisulphite sequencing (see Methods ) is also indicated between parentheses. Extensively methylated genes are the ones that have HMR from 500 bp upstream of 5′-end to 500 bp downstream of 3′-end. ( b ) Differential expression profiles of methylated genes. Boxplots show the ranges of R -values for each category of methylated genes. Genes with R -values below 12 are considered to be constitutively expressed [25] . Of the 20 densely methylated genes, a total of six were defined as being differentially expressed ( P -value of 0.029, Student t -test). Another seven genes were expressed in normal growth conditions (shown by RNA-seq data) whereas the remaining seven bona fide genes were not expressed in any of the tested conditions. Medians of the data are shown as black horizontal line in the box. Outliers are shown as whiskers. Numbers above each column show the number of genes in each category. Full size image We had previously estimated the degree of differential expression of P. tricornutum genes across 16 complementary DNA (cDNA) libraries by calculating the statistical significance of differential mRNA levels in specific conditions compared with random distribution (log likelihood ratio, R -value) [25] , [28] . Considering these criteria, constitutively expressed genes have low R -values (<12) while genes that are significantly overrepresented in specific growth conditions have high R -values (>12). We examined whether we could detect a correlation between gene methylation and R -value. We found that six genes with extensive HMR coverage have significantly increased R -values compared with genes with partial methylation and unmethylated genes ( Fig. 5b ). These observations suggest that the transcription of genes with extensive methylation is under tight control, that is, this gene population tends to be silenced and/or expressed only under specific conditions. For instance, gene model 13617, which encodes a serine/threonine protein kinase belonging to the eukaryotic core genes, shows zero FPKM under normal conditions but is specifically represented in the cDNA library prepared from P. tricornutum cells grown under silicate-deplete conditions ( Fig. 3f ). In contrast, genes showing partial methylation are more likely to be expressed constitutively. More specifically, body-methylated genes appear to be expressed at relatively low to moderate levels ( Supplementary Fig. S10 ). We also addressed whether we could detect a link between expression profiles and orthology groups but we found no significant correlation other than that methylated eukaryotic core genes were more likely to have lower R -values than the other categories ( Supplementary Table S6 ). In addition, methylated P. tricornutum -specific genes seem to be more tightly regulated as shown by their higher R -values, suggesting their potential importance in regulating gene expression under specific stress conditions ( Supplementary Table S6 ). As a first step to examine whether DNA demethylation is associated with the induction of gene expression, we selected genes that were both methylated in normal conditions and induced in response to nitrate limitation [25] . The methylation profile of these genes in nitrate-limiting conditions was then assessed by bisulphite sequencing, and a significant proportion (33 genes) were found to be demethylated and to display higher expression levels than in the normal nitrate replete conditions ( P -value=0.04; Student t -test, Pablo Rabinowicz, Maximo Rivarola, Jaysheel Bhavsar, Todd Creasy, Kimberly O'Brien, Naomi A. Sengamalay, Luke Tallon, Andrew Smith, Andy Allen; manuscript in preparation). This is illustrated in Supplementary Fig. S11 with gene model 39528 encoding carbamoyl phosphate synthase II and gene model 12902 that encodes a ferredoxin-dependent nitrite reductase. To assess more generally the function of the 326 methylated gene products, we performed a gene ontology (GO) analysis using hypergeometric test. Overall, we found that the methylated gene set is enriched ( P -value <0.00001, Student t -test) in GO categories such as ‘transferase activity,’ ‘transporter activity,’ ‘carbohydrate binding’ and ‘nutrient reservoir activity’ ( Supplementary Fig. S12a ). However, when comparing GO enrichment between sets of genes with different methylation profiles, we observed that, in contrast, the subset of genes with extensive methylation is enriched ( P -value=0.001, Student t -test) in ‘protein kinase’ and ‘signal transducer activity’ categories, which are evocative of regulatory and signalling functions ( Supplementary Fig. S12b ). Interestingly, when looking in more detail into metabolic pathways, we found that methylated genes are especially represented among genes predicted to be involved in pentose phosphate metabolism ( Supplementary Fig. S13a ). This pathway was reported previously to have unusual features in diatoms and to likely not be subject to regulation by thioredoxin, as is the case in other photosynthetic organisms [29] . DNA methylation may therefore have a role in the regulation of glucose turnover that produces NADPH and pentoses as essential backbones of nucleotides. When focusing on regulatory pathways, we found that at least three methylated genes were predicted to be involved in DNA mismatch repair, suggesting a role for DNA methylation in the maintenance of DNA integrity ( Supplementary Fig. S13b ). Methylation and non-autonomous Class II TEs In a previous study, we screened for autonomous TEs in the P. tricornutum genome using similarity-based approaches and searching for sequence structural characteristics specific of TEs. Here, in order to improve the quality of HMR mapping, we used the de novo repeat identification program Recon [30] and the tandem repeat finder program TRF [31] in an attempt to detect and annotate potentially unclassified or simple repeats in the genome. Most of the newly identified repeat loci lack HMRs. More specifically, although we were not able to classify most of the unknown repeats detected by Recon, we identified two families of non-autonomous Class II TEs with captured exons and analysed their m5C patterns individually. A first family, called R33, consists of six copies whose extremities are highly similar to the terminal inverted repeats of an inactivated MuDR-like element, and whose internal sequence contains an exon from the single-copy gene encoding 2-oxoglutarate dehydrogenase component E1 ( Supplementary Fig. S14a ). We found that none of the R33 copies nor the original gene overlap with HMRs, suggesting that R33 repeats are not targeted by the DNA methylation machinery, which is consistent with the inactive state of the cognate autonomous element. The second non-autonomous Class II family element, called R59, comprises four copies and appears to be linked to PiggyBac elements ( Supplementary Fig. S14b ). R59 has captured a fragment of exon from a single-copy gene encoding heat shock protein 70 ( HSP70 ). Interestingly, although PiggyBac elements in general were observed to be only moderately methylated, R59 displays much higher methylation levels. Even more unexpectedly, the original HSP70 gene (gene model 41417) also appears to be methylated, with HMR coverage extending out of the region of similarity with the captured region found in R59 ( Supplementary Fig. S14c ). This suggests that the presence of R59 copies in the genome may affect the epigenetic regulation of the HSP70 gene, which might ultimately impact its transcriptional regulation. In the work described herein, we have obtained the first genome-wide DNA methylation map of the nuclear genome of a stramenopile, namely the marine diatom P. tricornutum . Overall, DNA methylation in P. tricornutum is low, as previously reported using reversed-phase high-performance liquid chromatography [32] . It shows ~5% of global methylation with only 3.3% of genes methylated. This is lower than what is seen in mammals and in plants, such as Arabidopsis and rice, in which over 30% of genes are methylated [5] , [6] , [7] , [10] , but is similar to the marine tunicate Ciona intestinalis and the early-diverging land plant S. moellendorffii [20] . Consistent with previous studies [24] , we also found a significant enrichment of DNA methylation in TEs. Furthermore, we detected scarce DNA methylation in the intergenic space. The DNA methylation landscape of P. tricornutum is therefore reminiscent of the ‘mosaic’ landscapes observed in angiosperms with small genomes and invertebrates [33] , being composed of islands of HMRs surrounded by methylation-free regions. This first methylome from a stramenopile confirms the evolutionary conservation of gene-body methylation among eukaryotes [6] , [10] . Gene-body methylation was found to occur in various (epi)genomic contexts: in close proximity to TEs, in clusters of methylated genes and in single genes. In the case of methylated protein-coding genes that are flanked by repeats, we assume that methylation occurs through spreading from repeats. This indicates that, as seen in A. thaliana [26] , insertion of TEs can trigger the formation of heterochromatin around and within flanking genes. By contrast, methylated genes in repeat-free regions are likely to be methylated following a distinct and more specific mechanism. Methylated genes organized in clusters are evocative of coordinated transcriptional regulation, and examples were indeed found of methylated gene clusters whose genes displayed similar expression profiles ( Fig. 3f ). In all contexts, gene-body methylation was found almost exclusively in exons ( Supplementary Fig. S7 ), which is the case for most organisms investigated so far [6] , [9] . The functional annotation of body-methylated genes revealed that many encoded important metabolic activities, such as transferases, transporters, carbohydrate-binding proteins and other components involved in nutrient reservoir maintenance ( Supplementary Fig. S12a ). In contrast with such apparently housekeeping functions, genes that are extensively methylated tend to encode signalling components ( Supplementary Fig. S12b ). Furthermore, such genes tend to be silent under most conditions and differentially expressed only under specific conditions ( Fig. 5b ). We have observed previously that induction of the Blackbeard LTR-RT element in response to nitrate limitation is accompanied by loss of methylation [24] . In line with our previous observations, we report herein the demethylation of two genes involved in nitrate metabolism under nitrate starvation, a carbamoyl phosphate synthase and a nitrite reductase. It is therefore possible that in diatoms the perception of changing environments can trigger the hypomethylation of specific genes or TEs and release their transcriptional suppression, although genome-wide studies will be required to determine the extent of such processes. Of all P. tricornutum genes, ca. 30% (~3,000 genes) have been assigned a putative evolutionary origin, either from the ancestral exosymbiont, from one of the two algal endosymbionts, or by horizontal gene transfer from bacteria [19] , [20] . A further 25% are either specific to P. tricornutum or are specific to diatoms [20] , [25] . Such information provides an opportunity to examine whether distinct gene methylation patterns have been conserved during diatom evolution since they were acquired. We were unable to detect any such signatures. We further observed that bacterial genes tended not to be methylated, when compared with other gene classes ( Supplementary Fig. S9 ). Furthermore, bacterial genes are often associated with TE-rich regions ( Fig. 4 ). This may suggest that horizontal gene transfer of environmental DNA may be facilitated by TEs in a mechanism such as retroposition [29] , [34] , or perhaps that the insertion of such extraneous genes in repeat-rich regions may provide a probationary period in which their expression is attenuated and only released from repression gradually in case their effects may be deleterious. A further hypothesis would be that regions of the genome that have already inserted TEs are likely to be more permissive to horizontal gene transfer. Eukaryotes have evolved and/or retained different DNMT complements. Metazoans commonly encode DNMT1 and DNMT3 proteins, while higher plants additionally have plant-specific chromomethylase, and fungi have DNMT1, Dim-2, DNMT4 and DNMT5 (refs 35 , 36 ). Previous phylogenetic analysis suggests that the P. tricornutum genome encodes a peculiar set of DNMTs as compared with other eukaryotes [22] . DNMT1 appears to be absent, and in addition to DNMT3, diatom genomes also encode a DNMT5 protein as well as a bacterial-like DNMT. As DNMT5 is also found in other algae and fungi, we postulate that it was present in a common ancestor. Furthermore, structural, functional and phylogenetic data suggest that chromomethylase, Dim-2 and DNMT1 are monophyletic [35] , [36] . Therefore, we propose that the common ancestor of plants, unikonts and stramenopiles possessed DNMT1 (subsequently lost in diatoms), DNMT3 and probably also DNMT5 (lost in metazoans and higher plants). This evolutionarily important loss is supported by the absence of DNMTs in the stramenopile E. siliculosus [16] . In bacteria, cytosine methylation acts in the restriction-modification system. Thus, the function of a bacterial-like DNMT in P. tricornutum is unclear. Interestingly, this gene is conserved in the centric diatom Thalassiosira pseudonana, from which pennate diatoms such as P. tricornutum diverged ~90 million years ago. This implies that a diatom common ancestor acquired DNMT from bacteria after a horizontal gene transfer before the centric/pennate diatom split [18] . Conservation of this gene in diatoms over this length of time suggests that it is functional. It will therefore be of interest to uncover the roles of the different DNMTs present in P. tricornutum in processes such as maintenance and de novo DNA methylation as well as context specificities. Until now, bisulphite sequencing data indicate a clear CpG context preference in diatoms, although CHG and CHH contexts were also detected. P. tricornutum possesses an active small RNA-mediated silencing machinery [37] . This suggests that double-stranded RNAs are efficiently processed into small RNAs and that they are capable of guiding DNA methylation in an RNA-dependent DNA methylation (RdDM) fashion [38] , [39] , [40] . Furthermore, the presence of small RNAs was recently reported for both model diatom species T. pseudonana [41] and P. tricornutum [42] . Interestingly, in the latter, more than half of the highly methylated genes that are differentially expressed are targeted by small RNAs (for example, Fig. 3e ), suggesting that RdDM may have a role in the regulation of transcription of a subset of genes in diatoms, as recently inferred from studies of the atypical DNA methylation on some genes in A. thaliana [43] . Furthermore, we observed that the captured exon found in the R59 repeat is inserted in reverse orientation with respect to the PiggyBac backbone ( Supplementary Fig. S14 ). A scenario explaining the methylation found in the R59 repeat and the HSP70 gene could be that R59 is a source of transcripts with complementarity to HSP70 transcripts. The formation of double-stranded RNA duplexes may trigger their processing into small RNA that would target both R59 and HSP70 loci, and methylate them through RdDM. The cognate HSP70 gene was indeed found to be targeted by small RNAs ( Supplementary Fig. S14c ). RdDM may therefore represent an important mechanism of genome regulation in diatoms. In conclusion, the present work brings substantial information about the P. tricornutum methylome that enables analysis of methylation patterns and landscapes beyond animals, plants and fungi. P. tricornutum is of significant interest for such studies because it can be readily manipulated by reverse genetics. Unlike the other unicellular model organisms S. cerevisiae , Schizosaccharomyces pombe and Chlamydomonas reinhardtii , it has a small compact genome that displays all the key features of more complex genomes, such as DNA methylation, RNA interference and histone modifications. Furthermore, P. tricornutum has the peculiarity to be pleiomorphic as it can be found in the form of four different morphotypes: fusiform, oval, round and triradiate [44] . Significantly, morphotype transition occurs in response to specific environmental conditions such as salinity stress, temperature stress and nutrient limitation [44] , [45] . Therefore, P. tricornutum also constitutes an excellent model to study the basis of epigenomic reprogramming events that lead to morphological variations in response to external stimuli, for example, to assess the influence on adaptive evolutionary processes of the increased susceptibility of methylated genes to mutation. We therefore hope that our work on DNA methylation and its role in gene regulation in the diatom P . tricornutum will be the foundation for future work, and an exciting opportunity for comparative epigenomics and the elucidation of the dynamics of genome evolution in relation to the epigenetic regulation of gene expression. Culture conditions Cultures of P. tricornutum Bohlin clone Pt1 8.6 (CCMP2561) were grown in f/2 medium made with 0.2-μm-filtered and autoclaved seawater supplemented with f/2 vitamins and inorganic filter-sterilized nutrients. Cultures were incubated at 19 °C under cool white fluorescent lights at ~75 μmol m −2 s −1 in 12 h light:12 h dark conditions and maintained in exponential phase in semicontinuous batch cultures. DNA preparation To optimize the reproducibility and efficiency of methylated DNA exclusion, we modified the original protocol in a method called ‘Window McrBC Restriction’ (WMR; see Supplementary Methods ). Genomic DNA from three P. tricornutum cultures (biological replicates) was sonicated, size fractionated and incubated with McrBC enzyme (New England Biolabs). In negative controls, GTP, which is the cofactor required for McrBC activity, was replaced by water. Before hybridization, the DNA was further size selected as 500–700 nt fragments. Microarray hybridization and validation Microarray hybridization was performed according to Lippman et al . [23] , following NimbleGen’s ‘NimbleChip Arrays User’s Guide: DNA Methylation Analysis v2.0′ (Roche NimbleGen, Germany). NimbleGen 2.1M P. tricornutum tiling arrays were designed based on the JGI Phatr2 genome ( http://genome.jgi-psf.org/Phatr2/Phatr2.home.html ). A total of 2.1 million probes are represented on this array, which represents the entire+strand of the nuclear genome at 12-nt overlapping intervals. The average probe length was 56 nt. Both chloroplast and mitochondrial genomes, representing, respectively, 117 and 44 kb, were excluded from the array. NimbleGen provided design and probe annotation. We validated our methylation mapping approach by bisulphite sequencing of 28 randomly chosen loci including genes and TEs that are distributed at different locations in the genome ( Supplementary Table S1, S2 and S3 ). We included in the validation procedure one, two and three sparsely enriched probes to confirm that they had not been falsely discarded as a result of our strict filtering process. Altogether, these results enabled the validation of the mapping approach used for the identification of methylated regions. Furthermore, we used data from whole-genome bisulphite sequencing in normal and nitrate-limiting conditions (Pablo Rabinowicz, Maximo Rivarola, Jaysheel Bhavsar, Todd Creasy, Kimberly O'Brien, Naomi A. Sengamalay, Luke Tallon, Andrew Smith, Andy Allen; manuscript in preparation) to verify methylation in genes categorized as being methylated by McrBc-chip. RNA-seq preparation P. tricornutum clone Pt1 8.6 cells were harvested at exponential phase and total RNA was used for first-strand cDNA synthesis followed by double-strand cDNA using Mint Universal Kit from Evrogen (SK002). cDNA was used for non-directional cloning and cDNA library construction for Illumina sequencing by Beckman Coulter Genomics. Sequencing was performed with a read length of 75 bp and sequencing coverage of 1.5 Gb. Identification and analysis of methylated regions Statistically significant probe-bound regions (ChIP-enriched genomic regions) were detected using the RINGO package [46] in R Bioconductor. We used vsn normalization (variance stabilization) in RINGO, recommended for NimbleGen tiling microarray with multiple replicates. The strength of evidence for a ChIP-enriched site, that is, normalization, was assessed with a P -value cutoff of 0.02. The above procedure is to test every single probe for significant enrichment across all replicates (lfdr—local false discovery rate). Boundaries for methylated regions were defined as those with a minimum of three enriched overlapping probes, using a moving window of 50 bp. This is based on the array design, as each probe is on average 56 nt in length and tiled with 12 bp gap. We found at least 98,080 enriched probes, which amounts to 4.5% of probes covered. Normalization on the three biological replicates yielded robust consistency, which was statistically validated using a Student t -test and showed a Pearson R -value between 0.92 and 0.93 ( Supplementary Figs S15 and S16 ). Expression correlations with methylation were done using R -values derived from the EST sequences [25] and cDNA sequence data. Data processing, analysis and plotting were done using Python, R/Bioconductor and CIRCOS [47] (see Supplementary Methods ). A genome browser based on Gbrowse is available to explore this methylome data ( http://ptepi.biologie.ens.fr/cgi-bin/gbrowse/Pt_Epigenome ). Accession codes: The high-throughput sequencing data and microarray data have been deposited in NCBI’s Gene Expression Omnibus under GEO Series accession number GSE47947 . How to cite this article: Veluchamy, A. et al . Insights into the role of DNA methylation in diatoms by genome-wide profiling in Phaeodactylum tricornutum . Nat. Commun. 4:2091 doi: 10.1038/ncomms3091 (2013).